A biomimetic hybrid nanoplatform for encapsulation and precisely controlled delivery of theranostic agents Nanoparticles have demonstrated great potential for enhancing drug delivery. However, the low drug encapsulation efficiency at high drug-to-nanoparticle feeding ratios and minimal drug loading content in nanoparticle at any feeding ratios are major hurdles to their widespread applications. Here we report a robust eukaryotic cell-like hybrid nanoplatform (EukaCell) for encapsulation of theranostic agents (doxorubicin and indocyanine green). The EukaCell consists of a phospholipid membrane, a cytoskeleton-like mesoporous silica matrix and a nucleus-like fullerene core. At high drug-to-nanoparticle feeding ratios (for example, 1:0.5), the encapsulation efficiency and loading content can be improved by 58 and 21 times, respectively, compared with conventional silica nanoparticles. Moreover, release of the encapsulated drug can be precisely controlled via dosing near infrared laser irradiation. Ultimately, the ultra-high (up to ∼ 87%) loading content renders augmented anticancer capacity both in vitro and in vivo . Our EukaCell is valuable for drug delivery to fight against cancer and potentially other diseases. Chemotherapy has been widely used to treat cancer [1] . However, patients with chemotherapy often suffer from serious side effects of chemotherapeutic drugs [2] . Various nanoparticles have been explored for drug delivery to improve the safety and efficacy of chemotherapy [3] , [4] , [5] , [6] , [7] , [8] , [9] , [10] , [11] . However, regardless of their design, only part of the drug-laden nanoparticles can arrive at tumour in vivo and some can enter normal tissue [12] , [13] , [14] . Therefore, it is important to precisely control the drug release from nanoparticles specifically in tumour with minimal release in normal tissues. Another strategy for reducing the side effect of chemotherapy is to minimize the drug dose by combining it with other treatment modalities such as photothermal therapy (PTT, see Supplementary Note 1 for all acronyms) and photodynamic therapy (PDT) [15] , [16] , [17] . Moreover, the unique physicochemical properties of nanomaterials offer the opportunity to achieve both controlled drug release and the integration of different theranostic modalities into a single nanoplatform for combined therapy and in vivo imaging [18] , [19] , [20] , [21] . However, existing nanoparticles for this purpose often suffer from low drug encapsulation efficiency (EE) at high drug feeding ratios and minimal drug loading content (LC, usually less than ∼ 5%) in nanoparticle at any feeding ratios. The former entails significant waste of expensive chemotherapeutic drugs. The minimal drug LC makes it indispensable to use many times more exogenous materials (for making nanoparticles) than theranostic agents, which incurs significant safety concern [22] , [23] , [24] , [25] . To resolve these challenges, we developed a eukaryotic cell-like hybrid nanoparticle platform (EukaCell, with a phospholipid membrane, a cytoskeleton and a nucleus, although it does not have the cytoplasm) to achieve ultra-efficient encapsulation of doxorubicin hydrochloride (DOX) and indocyanine green (ICG) at both low and high drug feeding ratios for controlled delivery. DOX and ICG are widely clinically used chemotherapeutic drug and in vivo imaging agent, respectively. The DOX- and ICG-laden EukaCell enables combined therapy of chemo, PTT and PDT and allows for in vivo imaging. Characterization of EukaCell The EukaCell is made of fullerene (C60), mesoporous silica and phospholipid (1,2-dihexadecanoyl-sn-glycero-3-phosphocholine (DPPC)). Recently, C60 has attracted much attention for drug and gene delivery, PTT and PDT [26] , [27] , [28] . However, fullerene is still not widely used as of today because of its poor solubility in not only water but also commonly used organic solvents (for example, dimethylsulfoxide (DMSO) and dichloromethane) [29] . As illustrated in Fig. 1a , we embedded C60 fullerene in the centre of a mesoporous silica matrix to form the C60S nanoparticle. After modifying with (3-aminopropyl) trimethoxysilane (APTMS) to form the C60S-A nanoparticle, DPPC was fused on the surface of the C60S-A nanoparticle to produce the LC60S nanoparticle (that is, EukaCell). The resultant C60S and LC60S nanoparticles have high aqueous solubility, although fullerene easily aggregates in water ( Supplementary Fig. 1a ). This is further confirmed by shining a red laser beam through the solutions, which results in a discernible light track in the solutions of C60S and LC60S nanoparticles (asterisks in Supplementary Fig. 1b , the Tyndall effect) as a result of light scattering by the nanoparticles. Successful synthesis of the LC60S nanoparticles is further confirmed by the Fourier Transform Infrared spectroscopy (FTIR) data shown in Supplementary Fig. 2 . In addition, all the nanoparticles have a spherical and core-shell morphology and are ∼ 60 nm in diameter according to electron microscopy ( Fig. 1b,c and Supplementary Fig. 3 ). 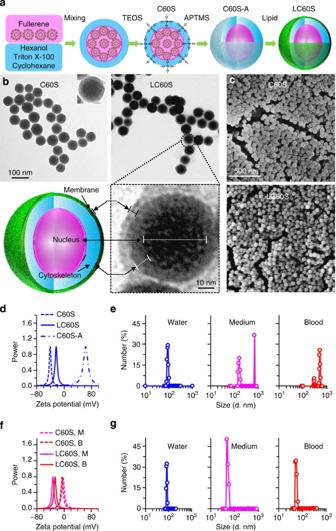Figure 1: Synthesis and characterization of biomimetic hybrid nanoparticles. (a) A schematic illustration of the procedure for preparing fullerene- (C60) embedded silica (C60S) nanoparticles, modifying the C60S nanoparticles with APTMS to form C60S-A nanoparticles, and further coating the C60S-A nanoparticles with phospholipids (DPPC) to produce LC60S nanoparticles. (b) Transmission electron microscopy images of the C60S and LC60S nanoparticles. Also shown is a zoom-in and schematic view of the LC60S nanoparticles to illustrate their eukaryotic cell-like configuration with a phospholipid membrane, a cytoskeleton of mesoporous silica and a nucleus of fullerene. (c) Scanning electron microscopy images of the C60S and LC60S nanoparticles showing their homogeneous size distribution. (d) The difference in surface zeta potential of C60S, C60S-A and LC60S nanoparticles indicating the successful coating of first positively charged APTMS and then negatively charged phospholipid on the surface of C60S nanoparticles. (e) Size distribution of C60S nanoparticles showing they form aggregates in both cell culture medium and the blood. (f) Surface zeta potential of C60S and LC60S nanoparticles in medium (C60S, M, and LC60S, M) and the blood (C60S, B, and LC60S, B) showing the LC60S nanoparticles stay negatively charged, whereas the C60S nanoparticles become nearly neutral. (g) Size distribution of LC60S nanoparticles showing their stability in water, culture medium and the blood. APTMS, (3-aminopropyl) trimethoxysilane; TEOS, tetraethyl orthosilicate. Figure 1: Synthesis and characterization of biomimetic hybrid nanoparticles. ( a ) A schematic illustration of the procedure for preparing fullerene- (C60) embedded silica (C60S) nanoparticles, modifying the C60S nanoparticles with APTMS to form C60S-A nanoparticles, and further coating the C60S-A nanoparticles with phospholipids (DPPC) to produce LC60S nanoparticles. ( b ) Transmission electron microscopy images of the C60S and LC60S nanoparticles. Also shown is a zoom-in and schematic view of the LC60S nanoparticles to illustrate their eukaryotic cell-like configuration with a phospholipid membrane, a cytoskeleton of mesoporous silica and a nucleus of fullerene. ( c ) Scanning electron microscopy images of the C60S and LC60S nanoparticles showing their homogeneous size distribution. ( d ) The difference in surface zeta potential of C60S, C60S-A and LC60S nanoparticles indicating the successful coating of first positively charged APTMS and then negatively charged phospholipid on the surface of C60S nanoparticles. ( e ) Size distribution of C60S nanoparticles showing they form aggregates in both cell culture medium and the blood. ( f ) Surface zeta potential of C60S and LC60S nanoparticles in medium (C60S, M, and LC60S, M) and the blood (C60S, B, and LC60S, B) showing the LC60S nanoparticles stay negatively charged, whereas the C60S nanoparticles become nearly neutral. ( g ) Size distribution of LC60S nanoparticles showing their stability in water, culture medium and the blood. APTMS, (3-aminopropyl) trimethoxysilane; TEOS, tetraethyl orthosilicate. Full size image The LC60S nanoparticles have a eukaryotic cell-like configuration ( Fig. 1b , sketch and zoom-in view) with a phospholipid membrane (DPPC), cytoskeleton (mesoporous silica) and nucleus (fullerene). The membrane is ∼ 5 nm thick, which is typical of a DPPC phospholipid bilayer [30] , [31] , [32] . The formation of the phospholipid membrane is further confirmed by the surface zeta potential of C60S, C60S-A and LC60S nanoparticles in deionized water. As shown in Fig. 1d , the zeta potential of C60S nanoparticles is negative at 22 °C (−41.4±2.3 mV). After modified with APTMS to form C60S-A nanoparticles, the zeta potential becomes positive (40.4±3.3 mV). After coating with the phospholipid bilayer, the zeta potential of the resultant LC60S nanoparticles returns to negative (−22.3±1.9 mV) and is similar to that of DPPC liposomes [33] . The phospholipid membrane is crucial to the high stability of the LC60S nanoparticles. Without it, the C60S nanoparticles aggregate into larger particles in both culture medium and blood, although they are stable in deionized water ( Fig. 1e ). The zeta potential of the C60S nanoparticles is almost zero in both medium and blood ( Fig. 1f ), suggesting the changes in their surface property contribute to their instability in the two biological solutions. In stark contrast, the LC60S nanoparticles are highly stable in both culture medium and blood with nearly unaltered negative zeta potential ( Fig. 1d,f ) and size distribution ( Fig. 1g ) in deionized water, culture medium and blood. Encapsulation of theranostic agents Remarkably, the LC60S nanoparticles can be used to encapsulate DOX in an ultra-fast and ultra-efficient manner at not only low but also high drug feeding ratios ( Fig. 2a–c and Supplementary Fig. 4 ). After mixing for only 10 min, ∼ 100% of the DOX can be encapsulated in the nanoparticles at a low drug feeding ratio of 1:20 (DOX/nanoparticle, often used for drug encapsulation with silica nanoparticles [34] , [35] ; Fig. 2a ). The EE is still 92.1% even for an unusually high drug feeding ratio of 1:0.5 with only 30 min of mixing, which is 58 times higher than that for nanoparticles made of silica (SiO 2 ) only ( Fig. 2b ). Moreover, the LC reaches 64.8±0.4%, which is ∼ 21 times higher than that of SiO 2 nanoparticles (3.1±0.8%, Fig. 2c ). It is worth noting that this ultra-high LC could minimize any potential toxicity of nanoparticles because the amount of nanoparticles needed for delivering the same amount of drug could be reduced by ∼ 21 times. With the further increase of the drug feeding ratio to 1:0.25, the LC improves to >71%. This efficient encapsulation of DOX by the LC60S nanoparticles is probably due to a double-interaction mechanism between DOX and the nanoparticles: the electrostatic interaction between DOX and silica [36] , [37] and the π–π stacking interaction between DOX and fullerene [38] , [39] . 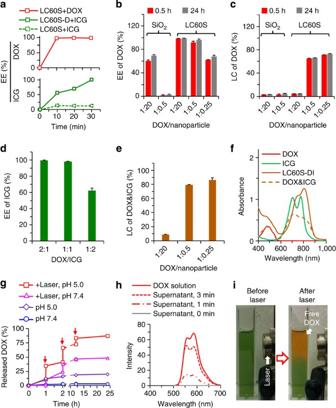Figure 2: Encapsulation and controlled release of theranostic agents. (a) Encapsulation efficiency (EE) of doxorubicin hydrochloride (DOX) and indocyanine green (ICG) by mixing the agents with nanoparticles for different times. The LC60S nanoparticles could encapsulate DOX efficiently but not ICG by simply mixing. However, by loading DOX first, the resultant DOX-laden LC60S (LC60S-D) nanoparticles could encapsulate ICG with an EE of∼100% by simply mixing for only 30 min. (b) EE and (c) loading content (LC) of DOX in LC60S and silica (SiO2) nanoparticles at different feeding ratios by simply mixing for 30 min and 24 h, showing the remarkably improved EE and LC of DOX in LC60S nanoparticles compared with the conventional SiO2nanoparticles. (d) The EE of ICG when mixed with LC60S-D nanoparticles at different ratios of DOX to ICG showing its dependence on the DOX content in the nanoparticles. (e) The total LC of DOX and ICG in LC60S-DI nanoparticles at different feeding ratios, showing efficient encapsulation of the theranostic agents. (f) Ultraviolet–visible absorbance of free DOX, free ICG, simple mixture of free DOX and ICG (DOX&ICG), and LC60S-DI nanoparticles. (g) DOX release from the LC60S-DI nanoparticles in phosphate-buffered saline (PBS) is pH dependent and can be precisely controlled with near infrared (NIR) laser irradiation. The arrows indicate laser irradiation at three different times. (h) Fluorescence intensity of free DOX solution and supernatant of LC60S-DI nanoparticle solution with the same DOX concentration after laser irradiation for 0, 1 and 3 min, further showing the drug release can be precisely controlled by dosing the NIR irradiation. (i) Pictures showing the colour change in the LC60S-DI (DOX/ICG=1:2) nanoparticles solution from green to yellowish after NIR laser irradiation due to the irradiation-induced release of DOX (red) from the nanoparticles. Before NIR irradiation, the red colour of DOX was quenched by the green colour of ICG. The unspecified ratios of DOX to LC60S nanoparticle and DOX to ICG for making the LC60S-DI nanoparticles were 1:20 and 1:1, respectively. All the NIR laser irradiation was for 1 min at 1.5 W cm−2. Figure 2: Encapsulation and controlled release of theranostic agents. ( a ) Encapsulation efficiency (EE) of doxorubicin hydrochloride (DOX) and indocyanine green (ICG) by mixing the agents with nanoparticles for different times. The LC60S nanoparticles could encapsulate DOX efficiently but not ICG by simply mixing. However, by loading DOX first, the resultant DOX-laden LC60S (LC60S-D) nanoparticles could encapsulate ICG with an EE of ∼ 100% by simply mixing for only 30 min. ( b ) EE and ( c ) loading content (LC) of DOX in LC60S and silica (SiO 2 ) nanoparticles at different feeding ratios by simply mixing for 30 min and 24 h, showing the remarkably improved EE and LC of DOX in LC60S nanoparticles compared with the conventional SiO 2 nanoparticles. ( d ) The EE of ICG when mixed with LC60S-D nanoparticles at different ratios of DOX to ICG showing its dependence on the DOX content in the nanoparticles. ( e ) The total LC of DOX and ICG in LC60S-DI nanoparticles at different feeding ratios, showing efficient encapsulation of the theranostic agents. ( f ) Ultraviolet–visible absorbance of free DOX, free ICG, simple mixture of free DOX and ICG (DOX&ICG), and LC60S-DI nanoparticles. ( g ) DOX release from the LC60S-DI nanoparticles in phosphate-buffered saline (PBS) is pH dependent and can be precisely controlled with near infrared (NIR) laser irradiation. The arrows indicate laser irradiation at three different times. ( h ) Fluorescence intensity of free DOX solution and supernatant of LC60S-DI nanoparticle solution with the same DOX concentration after laser irradiation for 0, 1 and 3 min, further showing the drug release can be precisely controlled by dosing the NIR irradiation. ( i ) Pictures showing the colour change in the LC60S-DI (DOX/ICG=1:2) nanoparticles solution from green to yellowish after NIR laser irradiation due to the irradiation-induced release of DOX (red) from the nanoparticles. Before NIR irradiation, the red colour of DOX was quenched by the green colour of ICG. The unspecified ratios of DOX to LC60S nanoparticle and DOX to ICG for making the LC60S-DI nanoparticles were 1:20 and 1:1, respectively. All the NIR laser irradiation was for 1 min at 1.5 W cm −2 . Full size image Drug release from the DOX-laden (LC60S-D) nanoparticles at pH 7.4 and 37 °C is minimal ( ∼ 4%) over 96 h in PBS ( Supplementary Fig. 5 ), which offers the opportunity to control the drug release specifically in tumour. We sought to employ heat that has been shown to disrupt the electrostatic interaction between DOX and silica [37] to control the drug release. To this end, we encapsulated ICG in the LC60S nanoparticles because ICG can generate heat under near infrared (NIR, ∼ 800 nm) laser irradiation [21] , [40] , [41] . The EE of ICG is low by simply mixing it with the LC60S nanoparticles ( Fig. 2a ). In stark contrast, when ICG is mixed with the DOX-laden LC60S (that is, LC60S-D) nanoparticles, the EE of ICG can be improved to 100% with 30 min mixing ( Fig. 2a ). The EE of ICG is ∼ 100% at the feeding ratios of 2:1 and 1:1 (DOX/ICG, Fig. 2d ), although it reduces to ∼ 60% at the feeding ratio of 1:2 (DOX/ICG). This suggests that one DOX molecule interacts with approximately one ICG molecule, which we attribute to the electrostatic interaction between the positively changed primary amine group in DOX and the negatively charged sulfonate group in ICG. With the feeding ratio of 1:0.5 for DOX/nanoparticle and 1:1 for DOX/ICG, the total LC in the DOX- and ICG-laden LC60S (that is, LC60S-DI) nanoparticle is ∼ 80%, and the EE of both DOX and ICG is more than 90% with 30 min mixing ( Fig. 2e ). The total LC can be further improved to ∼ 87% if the drug feeding ratio is 1:0.25. Successful encapsulation of both DOX and ICG in the LC60S-DI nanoparticles is further confirmed by the FTIR data shown in Supplementary Fig. 6 . It is worth noting that the C60S nanoparticles are also highly efficient for encapsulating DOX and ICG at both low (1:20) and high (1:0.5) feeding ratios of DOX (or ICG) to the nanoparticles ( Supplementary Fig. 7 ). The fullerene core and silica matrix are observable in the LC60S-DI nanoparticles made with low drug feeding ratios (for example, 1:20, Supplementary Fig. 8a ), but they are not clear in the LC60S-DI nanoparticles made with high drug feeding ratios (for example, 1:0.5, Supplementary Fig. 8b ). The latter is probably due to the high LC of agents that darken the whole space within the silica matrix. In addition, the high contrast induced by the darkened silica matrix makes the adjacent phospholipid membrane visible in the enlarged view of the nanoparticles ( Supplementary Fig. 8b ), even though the nanoparticle was not negatively stained with uranyl acetate, whereas the membrane is not evident in the LC60S-DI nanoparticles with a low drug LC without staining (the enlarged view in Supplementary Fig. 8a ). Moreover, a uniform size distribution of the nanoparticles is still evident at high drug feeding ratios ( Supplementary Fig. 8c ) and the LC60S-DI nanoparticles with both low and high LCs retain a negative zeta potential in deionized water, culture medium and blood ( Supplementary Fig. 9 ). After encapsulation in the LC60S-DI nanoparticles, the wavelength of the absorbance peak of ICG slightly increases with a redshift to 810 nm from 777 nm ( Fig. 2f ). However, if ICG and DOX are mixed directly in deionized water, the major absorbance peak undergoes slight blueshift. Moreover, the aqueous stability of ICG can be greatly improved by encapsulating it in the nanoparticles ( Supplementary Fig. 10 ). NIR laser controlled drug release We next investigated the in vitro release of DOX at 37 °C from the LC60S-DI nanoparticles. The drug release at pH 7.4 is negligible (<3%) after 24 h incubation, although it is faster at pH 5.0 ( Fig. 2g ). It is worth noting that the minimal drug release at pH 7.4 is not affected by the sequence of drug loading versus phospholipid coating ( Supplementary Fig. 11 ). Interestingly, the drug release is more sustained from the LC60S-DI (10.3±0.3, 1 h) than C60S-DI (27.7±0.4, 1 h, Supplementary Fig. 12 ) nanoparticles at pH 5.0, suggesting that the phospholipid membrane reduces the spontaneous drug release at the low pH. More importantly, the drug release can be triggered and precisely controlled by NIR laser irradiation ( Fig. 2g ), which we attribute to the laser irradiation-induced heating ( Supplementary Fig. 13 ) that disrupts the interactions between DOX and both fullerene and silica in the nanoparticles. To confirm this, we compared the drug release under six different conditions: LC60S-D nanoparticles with NIR irradiation for 3 min and LC60S-DI nanoparticles with heating in hot water bath at 45, 50, 60, 70 and 75 °C for 30 min or longer. As shown in Supplementary Fig. 14 , no drug release was triggered by either NIR irradiation of the LC60S-D nanoparticles in the absence of ICG or simply heating the nanoparticles at 45 °C in water bath. By contrast, heating at 50, 60, 70 and 75 °C in water bath triggers drug release. Moreover, the DOX release can be precisely controlled with the time (or dose) of NIR irradiation ( Fig. 2h ). The laser irradiation-controlled release of DOX is further confirmed by the change in colour of the aqueous solution of the LC60S-DI nanoparticles made from a low ratio of DOX to ICG (1:2; Fig. 2i ). Before laser irradiation, the red DOX is quenched by the green ICG in the nanoparticles. In summary, we have prepared eukaryotic cell-like nanoparticles for fast and efficient encapsulation of both DOX and ICG, and release of the encapsulated drug can be precisely controlled by dosing NIR irradiation, as illustrated in Supplementary Fig. 15 . In vitro anticancer capability The in vitro anticancer capability of the nanoparticle-encapsulated drug was investigated using PC-3 prostate and MDA-MB-231 breast cancer cells. We first incubated the cells with C60S, C60S-D and C60S-DI without a phospholipid membrane. As shown in Supplementary Fig. 16a,b , cytotoxicity of the nanoparticles with no drug is negligible. Without laser irradiation, the cytotoxicity of C60S-D and C60S-DI nanoparticles is similar to (for PC-3 cells) or slightly less than (for MDA-MB-231 cells) that of free DOX. More importantly, the cytotoxicity of C60S-DI to both PC-3 and MDA-MB-231cancer cells is greatly enhanced when combined with NIR irradiation. According to the confocal images shown in Supplementary Fig. 16c , free DOX mainly locates in the nuclei, whereas free ICG mainly stays in the cytoplasm. After treated with C60S-D or C60S-DI, DOX distributes in both the nuclei and cytoplasm, which indicates the drug was partially released from the nanoparticles. After laser irradiation, the increase of DOX fluorescence intensity in nuclei indicates more DOX was released from the nanoparticles. These data indicate that the drug release from C60S-DI nanoparticles in cells can be controlled by NIR irradiation. Similarly, with NIR irradiation, the LC60S-DI nanoparticles can effectively kill the cancer cells ( Fig. 3a,b ). Moreover, compared with free DOX and C60S-DI nanoparticles, the LC60S-DI nanoparticles without laser irradiation have significantly lower cytotoxicity ( Supplementary Fig. 17 ). These data suggest less DOX release from the LC60S-DI than C60S-DI nanoparticles during incubation with cells without NIR irradiation. This is consistent with the in vitro drug release study showing the phospholipid membrane can slow down the spontaneous drug release ( Fig. 2g and Supplementary Fig. 12 ). As a result, different from the C60S-DI treatment for which DOX distributes in both the nuclei and cytoplasm even without NIR irradiation ( Supplementary Fig. 16c ), the DOX fluorescence in cells treated with LC60S-DI nanoparticles without NIR irradiation is mainly in the cytosol ( Fig. 3c ). As DOX has to be in the nuclei and bind with DNA to induce cytotoxicity, this result indicates that the LC60S nanoparticle is a desirable platform for delivering chemotherapeutic drug with reduced side effects. Furthermore, when irradiated with NIR laser for 3 min, almost all DOX can be released from the LC60S-DI nanoparticles and bind to DNA in the nuclei ( Fig. 3c ), consistent with the in vitro drug release in PBS ( Fig. 2g–h ). Of note, there is significant overlap between the fluorescence of DOX, ICG and the green stain of late endosomes/lysosomes in both the PC-3 and MDA-MB-231 cancer cells after 3 h incubation with the LC60S-DI nanoparticles without NIR laser irradiation ( Supplementary Fig. 18 ), suggesting the cancer cells actively take up the nanoparticles via endocytosis. 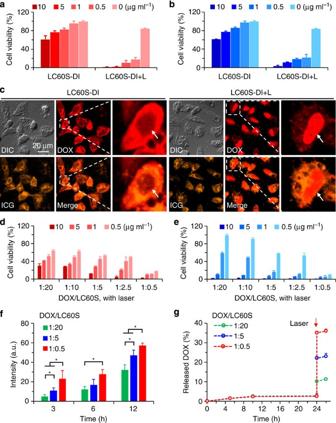Figure 3: Controlled drug release in cells and enhanced anticancer capacity with high drug LC. Viability of (a) PC-3 and (b) MDA-MB-231 cancer cells after treated with LC60S-DI nanoparticles at different concentrations without or with NIR laser (L) irradiation. (c) Confocal images showing the DOX and ICG delivered using LC60S-DI nanoparticles are mainly in the cytosol before NIR laser irradiation. With NIR laser irradiation, the enhanced delivery of DOX into the nuclei is evident probably due to the irradiation-induced release of DOX from the nanoparticles. The arrows indicate cell nuclei. Viability of (d) PC-3 and (e) MDA-MB-231 cancer cells after treated with LC60S-DI nanoparticles made at different drug feeding ratios (that is, different LCs) and NIR irradiation. The data show that the LC60S-DI nanoparticles with higher drug LC is more potent against both types of cancer cells at all the four doses. (f) The mean fluorescence intensity of DOX in PC-3 cells treated with LC60S-DI nanoparticles and laser irradiation showing a higher DOX LC results in significantly stronger DOX fluorescence in the cells. DOX (in LC60S-DI nanoparticles) concentration: 10 μg ml−1. Error bars represent±s.d. (n>50). *P<0.05 (Mann–WhitneyU-test). (g) Release of DOX from LC60S-DI nanoparticles in PBS showing that given the same DOX concentration (0.1 mg ml−1), NIR laser irradiation can induce more drug release from the nanoparticles with a higher drug LC. The unspecified ratios of DOX to LC60S nanoparticle and DOX to ICG for making the LC60S-DI nanoparticles were 1:20 and 1:1, respectively. The NIR laser irradiation was at 1.5 W cm−2for either 3 (a–c) or 1 min (d–g). Figure 3: Controlled drug release in cells and enhanced anticancer capacity with high drug LC. Viability of ( a ) PC-3 and ( b ) MDA-MB-231 cancer cells after treated with LC60S-DI nanoparticles at different concentrations without or with NIR laser (L) irradiation. ( c ) Confocal images showing the DOX and ICG delivered using LC60S-DI nanoparticles are mainly in the cytosol before NIR laser irradiation. With NIR laser irradiation, the enhanced delivery of DOX into the nuclei is evident probably due to the irradiation-induced release of DOX from the nanoparticles. The arrows indicate cell nuclei. Viability of ( d ) PC-3 and ( e ) MDA-MB-231 cancer cells after treated with LC60S-DI nanoparticles made at different drug feeding ratios (that is, different LCs) and NIR irradiation. The data show that the LC60S-DI nanoparticles with higher drug LC is more potent against both types of cancer cells at all the four doses. ( f ) The mean fluorescence intensity of DOX in PC-3 cells treated with LC60S-DI nanoparticles and laser irradiation showing a higher DOX LC results in significantly stronger DOX fluorescence in the cells. DOX (in LC60S-DI nanoparticles) concentration: 10 μg ml −1 . Error bars represent±s.d. ( n >50). * P <0.05 (Mann–Whitney U -test). ( g ) Release of DOX from LC60S-DI nanoparticles in PBS showing that given the same DOX concentration (0.1 mg ml −1 ), NIR laser irradiation can induce more drug release from the nanoparticles with a higher drug LC. The unspecified ratios of DOX to LC60S nanoparticle and DOX to ICG for making the LC60S-DI nanoparticles were 1:20 and 1:1, respectively. The NIR laser irradiation was at 1.5 W cm −2 for either 3 ( a – c ) or 1 min ( d – g ). Full size image Importantly, we found the LC60S-DI nanoparticles with higher drug LC could kill the cancer cells more effectively at the same drug dose under NIR laser irradiation ( Fig. 3d,e ), which is consistent with the stronger DOX fluorescence in cells treated with LC60S-DI nanoparticles with a higher drug LC after laser irradiation ( Fig. 3f and Supplementary Fig. 19 ). Presumably, this is because more DOX can be released from the LC60S-DI nanoparticles with a higher drug LC given the same dose of drug and NIR irradiation ( Fig. 3g ). Besides the chemo- and photothermal effect, we also examined the photodynamic capability of the LC60S, LC60S-D and LC60S-DI nanoparticles by checking the production of singlet oxygen in aqueous solutions ( Supplementary Fig. 20 ) and reactive oxygen species (ROS, including singlet oxygen) in cancer cells incubated with the nanoparticles ( Supplementary Fig. 21 ). The LC60S-DI nanoparticles can induce significantly more ROS production than the other nanoparticles after NIR irradiation and can be used to achieve tri-modal combination therapy of chemo, PTT and PDT. Biodistribution and controlled drug release in vivo We next investigated the biodistribution in mice of the LC60S-DI nanoparticles together with C60S-DI nanoparticles and the mixture of free DOX and ICG (DOX&ICG) at the same dose of the theranostic agents. As shown in Fig. 4a , at 2 h after intravenous injection, the ICG fluorescence was detectable over the whole animal body for all the three formulations with ICG. More importantly, stronger fluorescence in the tumour area is observable at this time only for mice treated with the LC60S-DI nanoparticles, indicating preferential accumulation of the LC60S-DI nanoparticles in tumour. The ICG fluorescence in the tumour area in mice treated with LC60S-DI nanoparticles further increases at 4 and 6 h. By contrast, no ICG fluorescence was detectable at 6 h or later in the tumour of mice treated with either DOX&ICG or C60S-DI nanoparticles. Furthermore, the ICG fluorescence could still be detected at 28 h in the tumour of mice treated with the LC60S-DI nanoparticles. 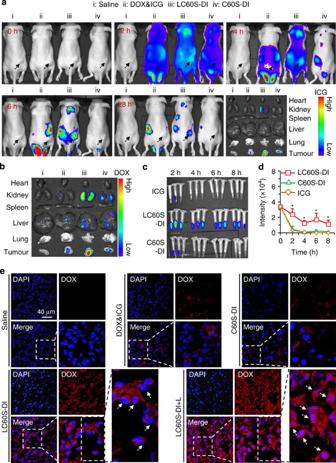Figure 4: Enhanced and controlled drug delivery to tumour. (a)In vivowhole animal imaging of ICG fluorescence at different times after intravenous injection via the tail vein in the forms of free DOX&ICG, LC60S-DI nanoparticles and C60S-DI nanoparticles together withex vivoimaging of ICG in tumour and five different organs collected after killing the mice at 28 h. The arrows indicate the locations of tumours in mice. (b)Ex vivoimaging of DOX fluorescence in the same tumour and organs. (c) Images and (d) the corresponding intensity of ICG fluorescence in blood drawn from the mice injected with LC60S-DI nanoparticles, C60S-DI nanoparticles and free ICG. The data indicate a significantly prolonged half-life of the LC60S-DI nanoparticles in blood circulation, compared with free ICG and C60S-DI nanoparticles. Error bars represent±s.d. (n=3). *P<0.05. (Kruskal–WallisHtest). (e) Fluorescence images of DOX in tumour of mice killed at 28 h post injection with saline, DOX&ICG, C60S-DI nanoparticles and LC60S-DI nanoparticles (with and without laser irradiation right before sacrificing the mice). The arrows indicate that for the treatment with LC60S-DI nanoparticles, NIR irradiation induces release of DOX from the nanoparticles so that it can enter the nuclei of cancer cells in tumourin vivo. Otherwise, the DOX stays with the nanoparticles in the cytosol with minimal cytotoxicity. The unspecified ratios of DOX to empty nanoparticle and DOX to ICG for making the DOX- and ICG-laden nanoparticles were 1:20 and 2:1, respectively. All the NIR laser irradiation was for 3 min at 0.7 W cm−2. Figure 4: Enhanced and controlled drug delivery to tumour. ( a ) In vivo whole animal imaging of ICG fluorescence at different times after intravenous injection via the tail vein in the forms of free DOX&ICG, LC60S-DI nanoparticles and C60S-DI nanoparticles together with ex vivo imaging of ICG in tumour and five different organs collected after killing the mice at 28 h. The arrows indicate the locations of tumours in mice. ( b ) Ex vivo imaging of DOX fluorescence in the same tumour and organs. ( c ) Images and ( d ) the corresponding intensity of ICG fluorescence in blood drawn from the mice injected with LC60S-DI nanoparticles, C60S-DI nanoparticles and free ICG. The data indicate a significantly prolonged half-life of the LC60S-DI nanoparticles in blood circulation, compared with free ICG and C60S-DI nanoparticles. Error bars represent±s.d. ( n =3). * P <0.05. (Kruskal–Wallis H test). ( e ) Fluorescence images of DOX in tumour of mice killed at 28 h post injection with saline, DOX&ICG, C60S-DI nanoparticles and LC60S-DI nanoparticles (with and without laser irradiation right before sacrificing the mice). The arrows indicate that for the treatment with LC60S-DI nanoparticles, NIR irradiation induces release of DOX from the nanoparticles so that it can enter the nuclei of cancer cells in tumour in vivo . Otherwise, the DOX stays with the nanoparticles in the cytosol with minimal cytotoxicity. The unspecified ratios of DOX to empty nanoparticle and DOX to ICG for making the DOX- and ICG-laden nanoparticles were 1:20 and 2:1, respectively. All the NIR laser irradiation was for 3 min at 0.7 W cm −2 . Full size image To confirm the aforementioned results of in vivo animal imaging based on ICG fluorescence, various organs were harvested for ex vivo imaging to check the distribution of ICG after killing the mice at 28 h. Only tumours from the LC60S-DI group show strong fluorescence of ICG ( Fig. 4a ). We further checked the distribution of DOX in the various organs. As shown in Fig. 4b , the DOX fluorescence is evident in the tumour of mice injected with LC60S-DI nanoparticles, whereas weak or no fluorescence is seen in the liver, heart, spleen and lung. In addition, DOX fluorescence is observable in the kidney, suggesting the LC60S-DI nanoparticles are cleared out of the body via the renal system after intravenous injection. By contrast, the DOX fluorescence intensity in all organs for the other two groups was weak or negligible. We attribute this to the short blood circulation time of the free agents and C60S-DI nanoparticles. As shown in Fig. 4c,d , free ICG disappears rapidly from blood circulation with a more than 70% reduction in fluorescence intensity within 2 h, as do C60S-DI nanoparticles. In contrast, the ICG fluorescence intensity in the blood of mice treated with LC60S-DI nanoparticles is significantly higher and more than half of the fluorescence intensity can retain at 8 h after injection. These data suggest that the LC60S-DI nanoparticles have a prolonged half-life in vivo , a desirable property of nanoparticles aimed for enhancing drug delivery. We further compared the biodistribution of LC60S-DI nanoparticles made from both low (1:20, DOX/nanoparticle) and high (1:0.5) drug feeding ratios. The results show that all the LC60S-DI nanoparticles can preferentially accumulate in tumour after intravenous injection ( Supplementary Fig. 22 ). The slight difference in the biodistribution of the nanoparticles made with the two different feeding ratios may be attributed mainly to the difference in (i) the total number of nanoparticles and (ii) LC of ICG in each nanoparticle given the same total dose of ICG administered intravenously. To examine the NIR irradiation-controlled drug release in vivo , mice either with or without NIR irradiation in the tumour area were killed at 28 h after drug injection and tumours were collected for cryo-sectioning and examining with fluorescence microscopy. As shown in Fig. 4e , the DOX fluorescence in tumours from LC60S-DI nanoparticle-treated mice is stronger than that of mice treated with C60S-DI nanoparticles or free DOX&ICG. Interestingly, the DOX fluorescence in tumour without laser irradiation is dominantly in the cytosol, which is similar to that in in vitro cells without laser irradiation ( Fig. 3c ). More importantly, with NIR irradiation, the presence of DOX in the nuclei is evident. These observations indicate minimal spontaneous drug release from the LC60S-DI nanoparticles and NIR irradiation can be used to precisely control the drug release in vivo , which should minimize the side effects of chemotherapy. In vivo antitumour capacity Last, we treated tumour-bearing mice with different drug formulations to understand the safety and efficacy of the LC60S-DI nanoparticle-based combination therapy of chemo, PDT and PTT. To check the biocompatibility of the LC60S nanoparticles, we mainly used LC60S-DI nanoparticles made from a low drug feeding ratio of 1:20 (DOX/nanoparticle) with a low drug LC (that is, to have much more materials than drug). No mice died during the course of the 4-week observation except for the C60S-DI group. After injection of C60S-DI nanoparticles, three out of six mice died during the first 2 days possibly due to aggregation of the C60S-DI nanoparticles in the blood ( Fig. 1e and Supplementary Fig. 23a,b ). Tumour growth for treatments of LC60S nanoparticles (blank), DOX&ICG, DOX&ICG with NIR irradiation (DOX&ICG+L) and C60S-DI nanoparticles with NIR irradiation (C60S-DI+L) is similar to that of saline control. The low efficacy of the C60S-DI+L treatment was probably due to the aggregation of the C60S-DI nanoparticles in the blood ( Fig. 1e and Supplementary Fig. 23b ), which prevents the nanoparticles from accumulating in tumour. A slight decrease in tumour volume was observed for the treatments of LC60S-D nanoparticles with NIR irradiation (LC60S-D+L) and LC60S-DI nanoparticles without NIR irradiation. Importantly, for the treatment of LC60S-DI nanoparticles with NIR irradiation (LC60S-DI+L), complete tumour destruction was observed in five out of six mice ( Fig. 5a,b ). The size and weight of the one remaining tumour in the LC60S-DI+L group are significantly less than that from the other aforementioned groups ( Fig. 5b,c ). Moreover, histological examination (haematoxylin and eosin (H&E) stain) revealed extensive necrosis in the remaining one tumour from the LC60S-DI+L group, whereas tumours from the other groups were more viable ( Fig. 5d ). More importantly, complete tumour destruction was observed in all the six mice treated with LC60S-DI nanoparticles made from a high drug feeding ratio of 1:0.5 (DOX/nanoparticle) with a high drug LC even though the time for laser irradiation was 2 min shorter (1 versus 3 min, Fig. 5a–c ). This is consistent with the in vitro cell viability study showing LC60S-DI nanoparticles with higher drug LC could induce higher cytotoxicity after NIR laser irradiation ( Fig. 3d,e ). 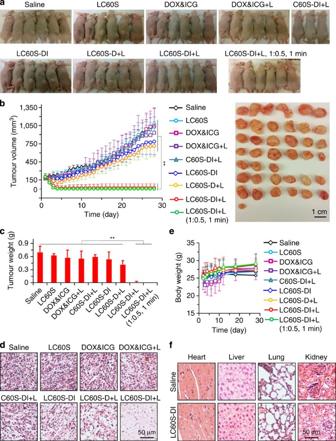Figure 5: Augmented safety and efficacy of cancer destructionin vivo. (a) Photographs of mice on day 28 after nine different treatments. (b) Growth curves of tumours in the mice together with images of the tumours collected on day 28 after killing the mice. Error bars represent±s.d. (n=3 for C60S-DI+L group,n=6 for other groups). **P<0.01. (Kruskal–WallisHtest). (c) Weight of the tumours collected after killing the mice on day 28. Error bars represent±s.d. (n=3 for C60S-DI+L group,n=6 for other groups). **P<0.01. (Kruskal–WallisHtest). (d) Representative images of histology (H&E) of the tumours collected on day 28. (e) Body weight of the mice with the various treatments showing no significant difference between them. (f) Histological (H&E) images of major organs collected on day 28 showing no evident systemic toxicity of the LC60S nanoparticles. The unspecified ratios of DOX to empty nanoparticle and DOX to ICG for making the DOX- and/or ICG-laden nanoparticles were 1:20 and 1:1, respectively. All non-specified NIR laser (L) irradiation was for 3 min at 0.7 W cm−2. The NIR irradiation was conducted at 12 h after intravenous administration of the various drug formulations. Figure 5: Augmented safety and efficacy of cancer destruction in vivo . ( a ) Photographs of mice on day 28 after nine different treatments. ( b ) Growth curves of tumours in the mice together with images of the tumours collected on day 28 after killing the mice. Error bars represent±s.d. ( n =3 for C60S-DI+L group, n =6 for other groups). ** P <0.01. (Kruskal–Wallis H test). ( c ) Weight of the tumours collected after killing the mice on day 28. Error bars represent±s.d. ( n =3 for C60S-DI+L group, n =6 for other groups). ** P <0.01. (Kruskal–Wallis H test). ( d ) Representative images of histology (H&E) of the tumours collected on day 28. ( e ) Body weight of the mice with the various treatments showing no significant difference between them. ( f ) Histological (H&E) images of major organs collected on day 28 showing no evident systemic toxicity of the LC60S nanoparticles. The unspecified ratios of DOX to empty nanoparticle and DOX to ICG for making the DOX- and/or ICG-laden nanoparticles were 1:20 and 1:1, respectively. All non-specified NIR laser (L) irradiation was for 3 min at 0.7 W cm −2 . The NIR irradiation was conducted at 12 h after intravenous administration of the various drug formulations. Full size image We did not notice any obvious side effect for the LC60S and LC60S-DI nanoparticles. Neither death nor significant drop of body weight was observed for the saline-, LC60S-, LC60S-DI-, LC60S-D+L- and LC60S-DI+L-treated mice ( Fig. 5e and Supplementary Fig. 23a ). The body weight of mice treated with free DOX did decrease during the first week after the drug treatment, although it was insignificant. This is because we treated the mice with the various drug formulations only once at a low dose (2.5 mg kg −1 body weight). In addition, no obvious damage to the major organs is observable in the H&E-stained slices of the organs ( Fig. 5f and Supplementary Fig. 24 ). Collectively, these data indicate the superior safety of the LC60S nanoparticles for delivering theranostic agents in vivo . For our in vitro cell imaging and viability studies, we temporarily replaced the drug-containing medium with pure medium (at room temperature) without any DOX or ICG during NIR laser irradiation. This is to avoid the effect and complication of the NIR laser irradiation-induced drug release from nanoparticles in the culture medium outside cells on the drug distribution and cell viability. According to Supplementary Fig. 13a , the temperature increase (Δ T ) in the pure culture medium without any ICG should be minimal. This, together with the facts that much more DOX distributes in the cell nuclei ( Fig. 3c ) and the cell viability significantly decreases ( Fig. 3a,b ) after the NIR laser irradiation for only 1 or 3 min at 1.5 W cm −2 , indicates that the temperature in the nanoparticles should be higher than 50 °C to trigger drug release in the in vitro cultured cells according to Supplementary Fig. 14 and much higher than the bulk medium temperature during the NIR laser irradiation. The bulk medium temperature should be no more than 4 °C higher than room temperature according to Supplementary Fig. 13a . In other words, the NIR laser irradiation-triggered drug release does not required a homogeneous high temperature in the bulk medium in vitro or bulk tumour tissue in vivo . The latter is supported by the data on the NIR laser irradiation-triggered drug release in vivo shown in Fig. 4e . This is because the bulk tissue temperature in tumour should be less than 50 °C according to the photothermal data shown in Supplementary Fig. 13a (together with the cooling effect of blood perfusion in vivo [42] ), under the condition of 0.7 W cm −2 NIR laser irradiation for up to 3 min with an ICG dose of 1.25 mg kg −1 body weight (which is equivalent to ∼ 1.25 μg ml −1 if we assume the tissue density is ∼ 1 kg l −1 , the same as that of water). It is worth noting that a mild hyperthermia (<50 °C) in tumour is desired to minimize overheating of normal tissue adjacent to the tumour because of heat dissipation from the tumour [42] , [43] , [44] , even though the temperature of the bulk tissue (or solution) with the LC60S-DI nanoparticles could also be raised to more than 50 °C for selective PTT by using a high concentration of ICG ( Supplementary Fig. 13b ). Indeed, we did not observe any overheating-induced carbonization or skin burning in mice treated with the NIR laser in this study. This nanoparticle (rather than bulk) temperature-triggered drug release is further supported by the in vitro cell viability and drug release data given in Fig. 3d–g , showing the LC60-DI nanoparticles with a higher drug LC (that is, higher ICG in each nanoparticle) could release more drug and kill more cancer cells than the nanoparticles with a lower drug LC (that is, lower ICG in each nanoparticle) even though the total doses of DOX/ICG and NIR laser irradiation are the same. Presumably, the temperature in each nanoparticle with a higher drug LC is higher under the same dose of NIR laser irradiation to trigger more drug release from the nanoparticle and kill more cancer cells. This should also contribute to the better tumour destruction in vivo with the LC60-DI nanoparticles made with a high drug feeding ratio of DOX to nanoparticle (1:0.5) given the same total doses of DOX/ICG and laser irradiation ( Fig. 5a–c ). In summary, both the EE and LC of theranostic agents are important parameters of multifunctional nanoparticles for drug delivery. To achieve high EE, low drug-to-nanoparticle feeding ratios have often been used for encapsulation, which in turn results in low drug LC. We have developed a eukaryotic cell-like nanoplatform or EukaCell, which can be used to achieve high EE ( ∼ 100%) and LC (up to ∼ 87%) of theranostic agents (DOX and ICG). As schematically illustrated in Supplementary Fig. 25 , release of the encapsulated drug can be precisely controlled using NIR laser irradiation to minimize the potential side effects. With the biomimetic (that is, eukaryotic cell-like) configuration, the EukaCell has a prolonged half-life and robust stability in blood circulation and can preferentially accumulate in tumour after intravenous injection. Ultimately, the drug-laden EukaCell exhibits superior safety and efficacy for cancer therapy. This study demonstrates the tremendous potential of our EukaCell for delivering theranostic agents to detect and treat cancer and potentially other diseases. Materials Cyclohexane, hexanol, Triton X-100, toluene, fullerene (C60), tetraethyl orthosilicate (TEOS), APTMS and ICG were purchased from Sigma-Aldrich. The phospholipid DPPC and cholesterol were purchased from Anatrace. DOX was purchased from LC Laboratories. The CCK-8 cell proliferation reagent was purchased from Dojindo Molecular Technologies. Fetal bovine serum (FBS) and penicillin/streptomycin were purchased from Invitrogen. The F-12K and DMEM cell culture media were purchased from American Type Culture Collection (ATCC). All other chemicals were purchased from Sigma unless specifically mentioned otherwise. Synthesis of nanoparticles Fullerene (C60) was encapsulated into the core of silica nanoparticles by a reverse microemulsion method. First, hexanol, Triton X-100, cyclohexane and deionized water were mixed together. A total of 2 ml of fullerene in toluene (2 mg ml −1 ) was then added into the mixture. Afterward, ammonium hydroxide (28 wt%, 60 μl) and TEOS (100 μl) were consecutively added and the sample was stirred at 800 r.p.m. using a mini-stir bar for 24 h at room temperature. Last, the sample was added into ethanol (30 ml) to stop the reaction. The final sample was centrifuged at 13,800 g for 10 min to obtain fullerene-embedded silica (that is, C60S) nanoparticles. After washing with deionized water and ethanol twice, the nanoparticles were dispersed in 3 ml of ethanol and 20 μl of APTMS (a silane coupling agent) was added. The mixture was stirred at 200 r.p.m. using a mini-stir bar for 12 h at room temperature to obtain the APTMS-coated C60S (that is, C60S-A) nanoparticles. Finally, the sample of C60S-A nanoparticles was mixed with DPPC liposomes and stirred for 5 h at room temperature to produce the phospholipid bilayer-coated C60S (that is, LC60S) nanoparticles. The LC60S nanoparticles were collected by centrifuging at 13,800 g for 10 min. The DPPC liposomes were prepared by hydrating a thin DPPC film. Briefly, 20 mg of DPPC and 5 mg of cholesterol were dissolved in 6 ml of the mixture of chloroform/methanol (2:1). The organic solvents were then removed by rotary evaporation at reduced pressure. The resultant dry film of DPPC deposited on the inner wall of the rotary flask was hydrated with 3 ml of phosphate-buffered saline (PBS, isotonic by default). After sonication for 2 min using a Branson 450 sonifier, the sample of DPPC liposomes ( ∼ 100 nm) was filtered through a 0.2-μm filter before mixing with the solution of C60S-A nanoparticles. Encapsulation and in vitro release of theranostic agents Encapsulation of the theranostic agents was conducted by mixing the agents with the nanoparticles at various feeding ratios of the agents to empty nanoparticles. The sequence of encapsulating DOX and ICG (dissolved in deionized water) was optimized in this study. Of note, unless specifically mentioned to be different (for high drug feeding ratios), the default ratio of DOX to empty nanoparticles for making DOX-laden nanoparticles was the commonly used value of 1:20. The default ratio of DOX to ICG for making the DOX- and ICG-laden nanoparticles was 1:1 and 2:1 for in vitro and in vivo studies, respectively. The former was based on our finding that one DOX molecule interacts approximately with one ICG molecule in the nanoparticles ( Fig. 2d ) to achieve maximum EE and LC of ICG. The latter with less ICG was used to achieve mild hyperthermia with a bulk tissue temperature less than ∼ 50 °C (that is, temperature increase less than ∼ 10 °C from body temperature, Supplementary Fig. 13a ) in tumour for in vivo studies to minimize damage to the surrounding normal tissue by heat dissipation. The EE of theranostic agents (DOX and/or ICG) using the nanoparticles was calculated using the following equation: where W Encapsulated represents the amount (in weight) of agents encapsulated into nanoparticles and was calculated using the following equation: where W Fed is the total amount of agents initially fed for encapsulation and W Non-encapsulated is the amount of agents remaining in the supernatant after centrifuging the sample. The amount of DOX and ICG in the supernatant was determined spectrophotometrically using a Beckman Coulter DU 800 ultraviolet–visible spectrophotometer based on their absorbance at 483.5 and 778 nm, respectively. The LC of theranostic agents was calculated with the following equation: where W Agent represents the amount of DOX and/or ICG in nanoparticles and W Total is the total amount of agent-laden nanoparticles including both the encapsulated agents and the non-agent materials for making the empty nanoparticles. To determine the long-term drug release in vitro , drug-laden nanoparticles (20–30 mg) were reconstituted in PBS (5 ml, at pH 5 or 7.4) and transferred into dialysis bags (MWCO: 20 kDa) that were placed in 30 ml of the same PBS solution at 37 °C and stirred at 110 r.p.m. using a mini-stir bar. At various times, 100 μl of the dialysate was collected and the remaining dialysate replenished with the same amount of fresh PBS. The concentration of the released DOX in the removed dialysate was determined using ultraviolet–visible spectrophotometry based on absorbance at 483.5 nm. For NIR laser irradiation-triggered drug release, the supernatant of the nanoparticle solutions was obtained by centrifuging at 13,800 g and analysed in the same way using ultraviolet–visible spectrophotometry. Characterization of empty and agent-laden nanoparticles The size and surface zeta potential of nanoparticles were assessed using a Brookhaven 90 Plus/BI-MAS dynamic light scattering instrument by dispersing the nanoparticles (1 mg ml −1 ) in deionized water, F-12K cell culture medium (containing 10% FBS by default) or plasma of mouse blood (10% in PBS). To prepare the blood plasma, fresh whole blood were collected into EDTA-coated centrifuge tubes and centrifuged for 10 min at 1,000 g and 4 °C. The supernatant was further centrifuged for 15 min at 2,000 g and 4 °C to deplete platelets and obtain blood plasma for experimental use. FTIR analysis of the nanoparticles was conducted using a Perkin Elmer Spectrum 100 FTIR spectrometer, for which samples were dried, ground in an agate mortar, thoroughly mixed with KBr at a ratio of ∼ 1:80 (nanoparticle:KBr) in weight and pressed into small discs at 10 tons for 5 min. The data were collected over 400–4,000 cm −1 . The morphology of nanoparticles was characterized using both transmission and scanning electron microscopy. For transmission electron microscopy studies, the nanoparticles were examined either directly (for C60S and agent-laden nanoparticles) or after negatively stained with uranyl acetate solution (2% (w/w), for empty LC60S nanoparticles) using an FEI Tecnai G2 Spirit transmission electron microscope. The scanning electron microscopy experiments were conducted by depositing 10 μl of aqueous solutions of the nanoparticles on a freshly cleaved mica grid and allowing them to dry for 60 min in the air. A thin film of Au was then sputtered onto the nanoparticles on the substrate. Samples were imaged with an FEI NOVA Nano400 scanning electron microscope. Detection of singlet oxygen production Deionized water, solution of LC60S nanoparticles, solution of LC60S nanoparticles irradiated with NIR laser, solution of LC60S-D nanoparticles, solution of LC60S-DI nanoparticles and solution of LC60S-DI nanoparticles irradiated with NIR laser were mixed with Singlet Oxygen Sensor Green reagent (Life Technologies) and fluorescence measurements were made using a Jasco FP-6200 spectrofluorometer with excitation and emission at 488 and 525 nm, respectively. Cell culture and in vitro cell viability Human prostate adenocarcinoma PC-3 cancer cells (ATCC) were cultured in F-12K medium supplemented with 10% FBS and 1% penicillin/streptomycin at 37 °C in a humidified 5% CO 2 incubator. Human breast adenocarcinoma MDA-MB-231 triple negative cancer cells (ATCC) were cultured in DMEM supplemented with 10% FBS and 1% penicillin/streptomycin at 37 °C in a humidified 5% CO 2 incubator. For cell viability studies, PC-3 and MDA-MB-231 cells were seeded overnight in 96-well plates followed by incubation with 100 μl of medium containing various drug formulations at different concentrations for 12 h. For the groups with NIR laser irradiation, the drug-containing medium was temporarily replaced with the same amount of pure medium (after three times of washing with the pure medium) at room temperature to avoid the effect and complication of NIR laser irradiation-induced drug release from nanoparticles outside cells and sticking of free DOX on culture plate on the cell viability studies. After applying the NIR laser irradiation, the pure medium was depleted and the drug-containing medium (maintained at 37 °C) was put back. All the samples were then further incubated with the various drug formulations for 12 h before determining the cell viability using the CCK-8 assay according to the instructions given by the manufacturer (Dojindo Molecular Technologies). In vitro imaging Cells were seeded onto collagen-coated cover glasses (Nunc, Thermo Fisher Scientific Inc.) at a density of 2 × 10 5 cells per well in six-well plate and grown at 37 °C for 12 h. The medium was then replaced with 1 ml of fresh medium containing different drug formulations to incubated with the cells at 37 °C for 3 h. For the groups with laser treatment, the drug-containing medium was replaced with the same amount of pure medium (after three times of washing with the pure medium) at room temperature and the cells were irradiated with NIR laser. The cells either with or without laser treatment were fixed in 4% paraformaldehyde for 15 min. The fixed cells attached on the cover glass were then washed with PBS for three times before mounting onto a glass slide with anti-fade mounting medium (Vector Laboratories) for examination using an Olympus FluoView FV1000 confocal microscope. Detection of ROS in cells Cells were cultured with different nanoparticles for 24 h. After NIR laser irradiation (if necessary), the cells were mixed with 25 μM dichloro-dihydro-fluorescein diacetate (Cell Bio Labs Inc.) for 45 min. Production of ROS was then detected quantitatively using a PerkinElmer VICTORX3 Multilabel microplate reader and qualitatively by fluorescence microscopy. Animals and xenograft tumours Athymic male NU/NU nude mice of 6-week-old were purchased from Charles River and maintained on a 16:8 h light–dark cycle. All procedures for animal use were approved by the Institutional Animal Care and Use Committee at The Ohio State University and all efforts were made to minimize animal suffering. To obtain xenograft of human prostate tumour in the nude mice, detached PC-3 human prostate cancer cells were suspended at 10 × 10 6 cells per millilitre in a mixture (1:1) of 1 × PBS and matrigel. A total of 1 × 10 6 cells in 100 μl of the mixture were injected subcutaneously at the dorsal side of the upper hindlimb of each 7-week-old mouse. In vivo imaging and biodistribution For in vivo imaging studies, after the tumour reached ∼ 5 mm in diameter, the mice were injected with 100 μl saline, a simple mixture of 100 μg DOX and 50 μg ICG in 100 μl saline, C60S-DI nanoparticles (DOX: 100 μg and ICG: 50 μg) in 100 μl saline or LC60S-DI nanoparticles (DOX: 100 μg and ICG: 50 μg) in 100 μl saline. In vivo fluorescence images were taken at 2, 4, 6 and 28 h after intravenous injection via the tail vein using a PerkinElmer IVIS instrument with an 831 nm filter to collect the fluorescence emission of ICG excited at 780 nm. After in vivo imaging, the mice were killed and the tumour, liver, kidney, lung, spleen and heart were removed and collected for further ex vivo fluorescence imaging of both DOX (with 560 nm filter and excitation at 488 nm) and ICG using the same IVIS instrument. To study the distribution of DOX (either as free drug or encapsulated in nanoparticles) in tumour cells after intravenous injection, tumours were collected and put in frozen with the Tissue-Tek (Sakura Finetek) O.C.T. Compound and Cryomold at −80 °C for 24 h. The tumours were then cut into slices of 10-μm thick using a cryo-microtome and transferred onto microscope slides. For 4,6-diamidino-2-phenylindole (DAPI) staining of cell nuclei, the slides were fixed in cold acetone for 10 min and then soaked in Tris buffer for 10 min before applying DAPI (1 μg ml −1 ) solution. After incubation at room temperature with DAPI for 10 min in the dark, the slides were examined using an Olympus FluoView FV1000 confocal microscope. In vivo antitumour efficacy and safety After tumours reached ∼ 5 mm in diameter, mice were randomly divided into nine groups and treated with 100 μl saline or LC60S nanoparticles, DOX&ICG (without or with NIR laser irradiation, 0.7 W cm −2 for 3 min, DOX: 2.5 mg kg −1 , ICG: 1.25 mg kg −1 body weight), C60S-DI nanoparticles with NIR laser irradiation (0.7 W cm −2 for 3 min, DOX: 2.5 mg kg −1 , ICG: 1.25 mg kg −1 body weight), LC60S-DI nanoparticles (DOX: 2.5 mg kg −1 , ICG: 1.25 mg kg −1 body weight), LC60S-D nanoparticles with NIR laser irradiation (0.7 W cm −2 for 3 min, DOX: 2.5 mg kg −1 body weight), LC60S-DI nanoparticles with NIR laser irradiation (0.7 W cm −2 for 3 min, DOX: 2.5 mg kg −1 , ICG: 1.25 mg kg −1 body weight) and LC60S-DI nanoparticles (feeding ratio of DOX/nanoparticle, 1:0.5) with NIR laser irradiation (0.7 Wcm −2 for 1 min, DOX: 2.5 mg kg −1 , ICG: 1.25 mg kg −1 body weight). A total of 100 μl saline was used as the carrier for all the drug formulations. The number ( n =6) of animals in each group was chosen to ensure statistical significance of the experimental data. The NIR laser irradiation was conducted at 12 h after the intravenous drug injection. During the NIR laser irradiation process, after every 1 min of irradiation, the tumour was allowed to spontaneously cool at room temperature for 30 s before the next irradiation to ensure that the overall tumour temperature was lower than ∼ 43 °C. Tumour growth was monitored every day. The tumour volume ( V ) was calculated as: V =0.5 × L × W 2 , where L is long diameter and W is short diameter determined using a caliper. The mice were euthanized at day 28 after the drug injection. Tumours, livers, lungs, hearts, spleens and kidneys were collected, formalin-fixed, paraffin-embedded and H&E stained for further histological analysis. Statistical analysis All data are reported as mean±standard deviation (s.d.) from at least three independent runs. The Kruskal–Wallis H -test and the Mann–Whitney U -test were used to assess the overall among-group and two-group differences, respectively. All statistical analyses were carried out with the IBM SPSS 22 software. How to cite this article: Wang, H. et al . A biomimetic hybrid nanoplatform for encapsulation and precisely controlled delivery of theranostic agents. Nat. Commun. 6:10081 doi: 10.1038/ncomms10081 (2015).